Programmable biofilm-based materials from engineered curli nanofibres The significant role of biofilms in pathogenicity has spurred research into preventing their formation and promoting their disruption, resulting in overlooked opportunities to develop biofilms as a synthetic biological platform for self-assembling functional materials. Here we present Biofilm-Integrated Nanofiber Display (BIND) as a strategy for the molecular programming of the bacterial extracellular matrix material by genetically appending peptide domains to the amyloid protein CsgA, the dominant proteinaceous component in Escherichia coli biofilms. These engineered CsgA fusion proteins are successfully secreted and extracellularly self-assemble into amyloid nanofibre networks that retain the functions of the displayed peptide domains. We show the use of BIND to confer diverse artificial functions to the biofilm matrix, such as nanoparticle biotemplating, substrate adhesion, covalent immobilization of proteins or a combination thereof. BIND is a versatile nanobiotechnological platform for developing robust materials with programmable functions, demonstrating the potential of utilizing biofilms as large-scale designable biomaterials. Advances in our understanding of bacterial systems in the past century have expanded the role of the microbe from being regarded solely as a health threat to being exploited as a genetically programmable factory for the production of biomolecules and chemicals. We view bacterial biofilms as embarking on a similar trajectory vis-à-vis functional advanced materials. The majority of bacteria in the natural world exist as biofilms: organized communities of cells ensconced in a network of extracellular matrix (ECM) composed of polysaccharides, proteins, nucleic acids and other biomolecular components [1] . This self-generated ECM protects bacteria from environmental rigours and mediates substrate adhesion, thus promoting microbial persistence and pathogenicity. Hence, the majority of biofilm research has focused on their eradication because of the negative roles biofilms play in clinical infection [2] . We envision instead the domestication of biofilms as a platform for programmable and modular self-assembling extracellular nanomaterials, with the bacterium serving as a living foundry for the synthesis of raw building blocks, their assembly into higher order structures upon secretion and the maintenance of the material as a whole over time. Although there has been some investigation into the use of biofilms for beneficial purposes such as energy generation [3] , wastewater treatment [4] and biotransformations [5] , [6] , these studies have primarily focused on altering the population of the biofilm microbial consortia rather than the ECM material itself. Another example is recent exciting work from the Wood group, in which they describe the design of synthetic genetic circuits that modulate the population balance in a dual-species biofilm to control biofilm formation and dispersal based on quorum-sensing [7] . Our approach to engineering the biofilm ECM material for practical applications focuses on the curli system–the primary proteinaceous structural component of E. coli biofilms. Curli are highly robust functional amyloid nanofibres with a diameter of approximately 4–7 nm that exist as extended tangled networks encapsulating the cells. Curli are formed from the extracellular self-assembly of CsgA, a small secreted 13-kDa protein. A homologous outer-membrane protein, CsgB, nucleates CsgA assembly and also anchors the nanofibres to the bacterial surface. Detached curli fibres can also exist as non-cell-associated structural components of the ECM. The curli genes exist as two divergently transcribed operons ( csgBAC and csg DEFG ) [8] , whose seven products mediate the structure (CsgA), nucleation (CsgB), processing (CsgE, F), secretion (CsgC, G) and direct transcriptional regulation (CsgD) of curli nanofibres. The curli system exhibits numerous features that make it an ideal platform for the type of materials engineering by way of synthetic biology that we envision. First, as the curli nanofibre is composed primarily from the self-assembly of one small protein, it presents a tractable entry point towards creating a large diversity of biofilm extracellular matrices with conventional genetic engineering methods. In contrast, it would be more difficult to engineer the exopolysaccharide component of biofilms, as polysaccharide synthesis is often tied to multi-step pathways with a limited tolerance for chemically diverse monomers compared with the protein synthetic machinery. Second, the functional amyloid fibres formed by CsgA are extremely robust, being able to withstand boiling in detergents [9] and extended incubation in solvents, increasing their potential utility in harsh environments. Similar amyloid nanofibres have been shown to have a strength comparable to steel and a mechanical stiffness comparable to silk [10] , suggesting that biofilms with high amyloid content would be able to withstand mechanically demanding environments. Third, functional amyloid fibrils are abundant in many naturally occurring bacterial biofilms and can constitute up to 10–40% of the total biovolume of a biofilm [11] , indicating that curli can be artificially engineered to comprise a significant portion of the biofilm. In addition, although analogous extracellular functional amyloids are produced by many bacteria, the curli system is currently the best studied and is native to the canonical model bacterium E. coli , making it an attractive starting platform for the development of engineered materials. Finally, recent findings have shown that the curli system can be used to efficiently export natively unfolded polypeptides and was capable of producing a functional camelid antibody fragment, suggesting that the curli system can be used in a broad and modular way for the display of various functional peptides throughout the E. coli biofilm ECM [12] , [13] . Here we show a Biofilm-Integrated Nanofiber Display (BIND) system to enable precise genetic programming of the E. coli biofilm ECM material by fusing functional peptide domains onto the CsgA protein. We demonstrate that the chimeric CsgA variants are secreted by the native cellular export machinery and assemble into networks of curli fibres resembling the wild-type system. We also show that this technique is compatible with a wide range of peptide domains of various lengths and secondary structures. Last, we demonstrate that the peptide domains maintain their function after secretion and assembly and confer artificial functions to the biofilm as a whole. Very recently, Chen et al . [14] have demonstrated a parallel curli-based system similar to our BIND concept, and show controlled multiscale patterning of single amyloid fibres and the use of engineered curli for the organization of gold nanoparticles and quantum dots for nanoelectronics applications. Herein, we expand on the functions that can be engineered into curli nanofibres by demonstrating three broad functions that we artificially introduce into the E. coli biofilm ECM: inorganic nanoparticle templating, specific abiotic substrate adhesion and the site-specific covalent immobilization of an arbitrary functionalized recombinant protein. Determination of an optimal peptide fusion site for CsgA The BIND strategy consists of reprogramming the self-assembling amyloid component of E. coli biofilms using genetic fusions of CsgA to functional peptides ( Fig. 1 ). To determine suitable fusion points to append peptides to CsgA, we generated a library ( Fig. 2a ) consisting of N- and C-terminal fusions to a test peptide domain designated MBD (for Metal Binding Domain). The MBD peptide has been shown to bind strongly to stainless steel surfaces and is derived from a segment of the Pseudomonas aeruginosa type IV pilus [15] . CsgA-terminal fusions were chosen to allow for the integration of both linear and circularly constrained peptides. Three variants were prepared for each terminus with varying glycine-serine flexible linker lengths. We used the standard amyloid-staining colorimetric dye, Congo Red [16] (CR), to determine the extent of curli production for the various mutants. The csgA variants were expressed in the model E. coli csgA deletion strain LSR10 (MC4100::Δ csgA ) that retains the remaining curli processing machinery under native regulation [8] . This strain has previously been used in numerous studies on the curli system as it has been shown to not produce flagella, cellulose or lipopolysaccharide O -polysaccharides, making it ideal for curli complementation studies [17] , [18] , [19] . Thus, LSR10 was chosen as a model strain for developing BIND in part because any colorimetric signal obtained from CR staining could be attributed to the presence of heterologously produced curli fibres, as opposed to cellulose or other biofilm components that may have the capability to bind CR nonspecifically [20] . Likewise, any extracellular fibres observed by transmission electron microscopy (TEM) and scanning electron microscopy (SEM), ultrastructural characterization can be attributed solely to the self-assembly of heterologously engineered CsgA fusion mutants. 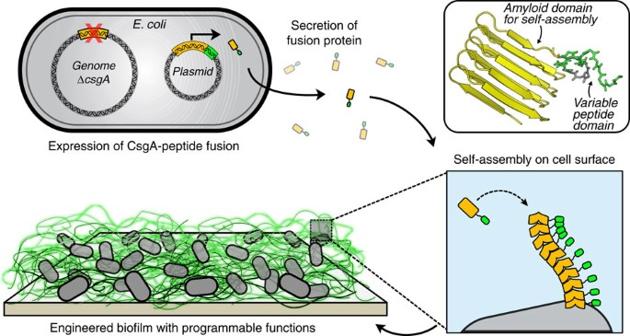Figure 1: Genetic programming and modularity of the BIND system. In the BIND platform,ΔcsgAcells heterologously express and secrete fusion proteins consisting of an amyloidogenic domain (CsgA, shown in orange) and a functional peptide domain (green). This secreted fusion protein self-assembles into an extracellular network of amyloid nanofibres that are anchored onto the cell surface, resulting in a biofilm material with programmed non-natural functions. A three-dimensional protein model is shown of the self-assembling and functional peptide domains, using homology model protein threading of the CsgA sequence onto an AgfA structure. An example peptide domain, SpyTag (seeTable 1), is shown in green and the six-residue flexible linker in grey. The peptide structure was predicted using PepFold and all structural manipulation performed in PyMol. Figure 1: Genetic programming and modularity of the BIND system. In the BIND platform, ΔcsgA cells heterologously express and secrete fusion proteins consisting of an amyloidogenic domain (CsgA, shown in orange) and a functional peptide domain (green). This secreted fusion protein self-assembles into an extracellular network of amyloid nanofibres that are anchored onto the cell surface, resulting in a biofilm material with programmed non-natural functions. A three-dimensional protein model is shown of the self-assembling and functional peptide domains, using homology model protein threading of the CsgA sequence onto an AgfA structure. An example peptide domain, SpyTag (see Table 1 ), is shown in green and the six-residue flexible linker in grey. The peptide structure was predicted using PepFold and all structural manipulation performed in PyMol. 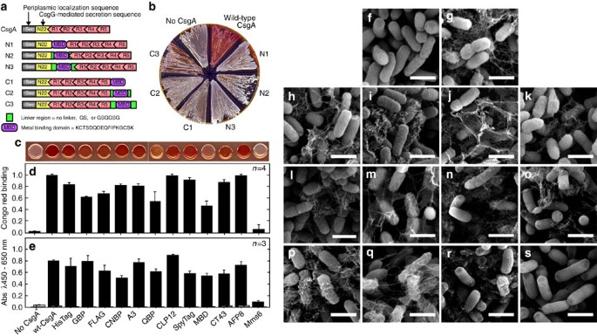Figure 2: Genetic engineering of the BIND platform. (a) A library of CsgA fusion mutants in which the MBD peptide insert (purple) was placed at the N- or C-terminus of the curlin repeat domains (red) and flanked by a six-residue linker, two-residue linker or no linker (green). (b) The MBD insert library was transformed into LSR10 (MC4100,ΔcsgA) cells and streaked onto YESCA-Congo Red induction plates. Red staining indicates amyloid production. (c) A representative set of culture spots of a BIND library consisting of 12 various functional peptides on YESCA-Congo Red induction plates (enumerated inTable 1). (d) Quantitative Congo Red values were obtained from quadruplicate YESCA-CR spotted cultures using intensity quantification (ImageJ) measurements of the relative amyloid produced for each CsgA-peptide fusion, normalized to wild-type CsgA. Standard error is shown. (e) Whole-cell filtration ELISA using an anti-CsgA antibody (black bars); secondary antibody–only controls are shown as grey bars. Each experiment was performed in triplicate and standard error is shown. FE-SEM images of the peptide fusion BIND library transformed into LSR10 (MC4100, ΔcsgA) cells with no CsgA (f), wild-type CsgA (g) and the BIND peptide panel (seeTable 1): HIS (h), GBP (i), FLAG (j), CNBP (k), A3 (l), CLP12 (m), QBP1 (n), SpyTag (o), MBD (p), CT43 (q), AFP8 (r) and Mms6 (s). All scale bars are 1 μm. Full size image Figure 2: Genetic engineering of the BIND platform. ( a ) A library of CsgA fusion mutants in which the MBD peptide insert (purple) was placed at the N- or C-terminus of the curlin repeat domains (red) and flanked by a six-residue linker, two-residue linker or no linker (green). ( b ) The MBD insert library was transformed into LSR10 (MC4100, ΔcsgA ) cells and streaked onto YESCA-Congo Red induction plates. Red staining indicates amyloid production. ( c ) A representative set of culture spots of a BIND library consisting of 12 various functional peptides on YESCA-Congo Red induction plates (enumerated in Table 1 ). ( d ) Quantitative Congo Red values were obtained from quadruplicate YESCA-CR spotted cultures using intensity quantification (ImageJ) measurements of the relative amyloid produced for each CsgA-peptide fusion, normalized to wild-type CsgA. Standard error is shown. ( e ) Whole-cell filtration ELISA using an anti-CsgA antibody (black bars); secondary antibody–only controls are shown as grey bars. Each experiment was performed in triplicate and standard error is shown. FE-SEM images of the peptide fusion BIND library transformed into LSR10 (MC4100, Δ csgA ) cells with no CsgA ( f ), wild-type CsgA ( g ) and the BIND peptide panel (see Table 1 ): HIS ( h ), GBP ( i ), FLAG ( j ), CNBP ( k ), A3 ( l ), CLP12 ( m ), QBP1 ( n ), SpyTag ( o ), MBD ( p ), CT43 ( q ), AFP8 ( r ) and Mms6 ( s ). All scale bars are 1 μm. Full size image The CR staining assay of the MBD insertion library indicated only the C3 fusion site with the longest C-terminal linker between CsgA and MBD was able to form an appreciable amount of amyloid fibres ( Fig. 2b ), albeit at a lower amount than the wild-type CsgA. It is possible that the N-terminal fusions had impaired secretion as a result of their proximity to the CsgG-specific export recognition sequence. Ultrastructural characterization by SEM ( Fig. 2n ) and TEM ( Supplementary Figs 1k and 2j ) of the C3 mutant curli nanofibres confirmed that they exhibited morphology similar to that of the wild-type CsgA fibres. CsgA peptide fusions retain amyloid self-assembly function Having identified the C3 fusion site as suitable for the display of peptides on the CsgA scaffold, we next created a library of 12 various peptide domain fusions to test the effect of peptide length and structure on secretion and assembly. The library members, detailed in Table 1 , range in length from 7–59 amino acids and encode a wide variety of functions such as binding to various inorganic substrates (GBP, CNBP, QBP, MBD and AFP8), nucleation of mineral and metallic nanostructures (A3, CLP12, CT43 and Mms6), and a highly specific catalytic interaction with a protein (SpyTag) [15] , [21] , [22] , [23] , [24] , [25] , [26] , [27] , [28] , [29] , [30] , [31] . Each peptide domain was cloned as C-terminal fusions to CsgA with an intervening six-amino-acid flexible linker ( Table 1 ) and these plasmids were expressed in LSR10 cells to produce 12 different BIND biofilms. Table 1 Functional peptide library incorporated into BIND. Full size table Relative differences in curli production between library members were monitored by measuring the staining intensity of transformants spotted on CR plates ( Fig. 2c,d ). CR binding is highly indicative of amyloids, providing a qualitative assessment of CR-binding extracellular material. These CR assays indicate that small peptide fusions may be tolerated by the curli export machinery and could successfully assemble into extracellular amyloid networks as evidenced by greater CR staining of all peptide fusions compared with the empty plasmid control. The only mutant for which there was no positive CR staining was the 59-amino-acid Mms6 protein domain, confirming previous findings that polypeptides with long sequences or inherent structure may not be exported efficiently through the CsgG outer membrane transporter, which has a pore size of 2 nm (ref. 32 ). As CR is also known to bind to other molecules in addition to amyloids, a more specific assessment of the amyloid-nature of proteins is provided from birefringence of the CR-stained material observed under polarized light [33] , [34] , [35] . 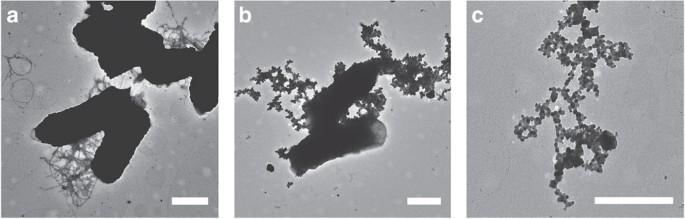Figure 3: Nanoparticle templating by BIND. Silver nanoparticles were templated by A3-BIND biofilms incubated in aqueous AgNO3. Representative TEM micrographs demonstrate that PHL628 ΔcsgAcells producing wild-type CsgA (a) show no nanoparticle templating, whereas A3-BIND (b) templates nanoparticles after incubation in 147 mM AgNO3for 4 h. (c) A higher magnification of the Ag nanoparticles organized on A3-BIND nanofilaments is shown. All scale bars are 0.5 μm. Cell masses of the BIND colonies from YESCA-CR plates were analysed by polarization microscopy ( Supplementary Figure 3 ). Most of the BIND variants exhibited birefringence characteristic of amyloids, although the intensity of the birefringence varied. The no curli control and Mms6-BIND samples showed no birefringence, as expected. Surprisingly, the CLP12- and QBP-BIND samples showed very low levels of birefringence, although they have high levels of CR binding. We posit that this is due to the amyloid fibres being highly dispersed or the presence of these peptides altering the binding mode of the CR such that birefringence is suppressed. To validate that the CR staining is due to the presence of extracellular materials containing CsgA, such as curli fibres, we performed whole-cell filtration ELISAs using anti-CsgA antibodies ( Fig. 2e ). Only extracellular material composed of CsgA and retained by the 0.22-μm filter would generate a CsgA-positive signal. The whole-cell ELISA data correlate with the CR staining results, confirming that CsgA-containing proteins are present extracellularly and are present as high-molecular-weight assemblies. However, the ELISA data does not discriminate intact fusion proteins from possible breakdown products. To investigate the possibility that these extracellular amyloids are due to the secretion and assembly of partially proteolysed CsgA fusion proteins and not the desired full-length CsgA fusion proteins, we isolated the extracellular fractions of induced BIND colonies and subjected this fraction to SDS solubilization. The SDS-insoluble fraction was collected by ultracentrifugation and dissolved in hexafluoroisopropanol (HFIP) to disassemble the curli fibres into their monomeric components. matrix-assisted laser desorption/ionization (MALDI)–time of flight (TOF)/TOF analysis of the resulting dissolved samples confirms the presence of mass peaks that correlate with the predicted mature CsgA fusion proteins in all of the samples except for the no curli control and the Mms6-BIND sample ( Supplementary Figs 4 ). Although this does not rule out potential proteolysis events, it does demonstrate that the extracellular fraction contains, to some degree, intact CsgA fusion proteins that are in an SDS-insoluble state, suggesting that the desired proteins are assembled into amyloid structures. It is possible amorphous extracellular aggregates could contribute to the CR-binding, whole-cell ELISA and MALDI results. To further confirm the presence of curli nanofibres and rule out unstructured extracellular aggregates in the BIND biofilms, we extensively analysed the ultrastructure of the curli biofilms using SEM ( Fig. 2f–s ) and TEM ( Supplementary Fig. 1 ). For the CR-positive transformants, fine nanofibres associated with the cells were observed, which are similar in morphology to wild-type CsgA. High-magnification TEM analysis of the BIND nanofibres revealed that they have a diameter of 4–7 nm, consistent with that previously reported for curli nanofibres [36] ( Supplementary Fig. 2 ). The BIND nanofibres displayed a characteristic tangled morphology and were observed to be closely associated with the cell surface or sometimes existing as free-floating masses. No extracellular fibres were observed for either the empty plasmid control or the Mms6-BIND biofilm ( Fig. 2f,s and Supplementary Fig. 1a,n ), corroborating the lack of CR staining and whole-cell ELISA signals for these samples. We additionally performed immunogold labelling of the BIND biofilms producing the CsgA-FLAG fusion protein, using an anti-FLAG antibody. The immunogold TEM images show localization of the gold nanoparticles to the curli fibre tangles, confirming both the presence and accessibility of the FLAG peptide domain ( Supplementary Fig. 5 ). In sum, the CR staining and CR birefringence experiments demonstrate the presence of extracellular amyloid, the whole-cell filtration ELISA data indicate that the CsgA fusions are present as extracellular assemblies, the MALDI analysis confirms the presence of SDS-insoluble extracellular material correlating in mass to the expected fusion proteins and the electron microscopy imaging of the BIND biofilms provides ultrastructural verification of the nanofibrillar morphology of the BIND ECM. Thus, peptides of arbitrary sequence and function can be efficiently displayed as C-terminal fusions to CsgA for extracellular self-assembly into functionalized curli nanofibres. The true value of the BIND system is in its ability to perform as an expansive interfacial biomaterial whose function can be genetically programmed in a modular manner. As a demonstration of some of these capabilities, we selected three peptides from Table 1 (FLAG, A3, MBD and SpyTag) with diverse functions and tested their ability to introduce these new functions into curli-producing biofilms. Specifically, we investigated the ability to programme biotemplating of inorganic nanoparticles (A3), enhanced adhesion to abiotic surfaces (MBD) and covalent immobilization of full-length proteins into the BIND biofilms (SpyTag). We also examined the generation of multifunctional BIND biofilms (FLAG and SpyTag). For these functional studies, we chose a different cell strain as a chassis for robust curli production, a previously developed csgA deletion mutant of the E.coli K-12 strain PHL628 (ref. 37 ). Although they also produce cellulose, which made them unsuitable for the initial characterization of the BIND platform, the PHL628 (MG1655 malA-Kan ompR234 ) cells are superior to the LSR10 strain for curli production because of a single point mutation in the OmpR protein, which enhances expression of the entire curli operon by ~3.5 × , resulting in substantial amounts of curli production [38] . This phenotype is ideal for generating expansive amyloid-rich ECM for functional analysis; plasmid-based overexpression of heterologous BIND variants in a Δ csgA PHL628 knockout mutant (hereafter referred to just as PHL628) is likely to prevent accumulation of the fusion proteins intracellularly by providing a high basal production of the proteins required for efficient processing and secretion of the CsgA fusions. Expression of the entire BIND peptide library in PHL628 cells resulted in similar relative curli production patterns as determined by CR binding in comparison to the LSR10 strain ( Supplementary Fig. 6 ). We also performed whole-cell filtration ELISAs on the FLAG-, A3-, SpyTag- and MBD-BIND biofilms to show that the CsgA protein is exported and assembles into a high-molecular-weight extracellular material ( Supplementary Fig. 7a,c,e,g ). Furthermore, MALDI-TOF/TOF analysis of the SDS-insoluble purified extracellular material shows mass peaks that correspond to that of the expected fusion proteins, suggesting that they are present and unproteolysed as amyloid fibrils in the ECM ( Supplementary Fig. 7b,d,f,h ). Silver nanoparticle templating onto A3 BIND nanofibres Engineered peptides functionalized onto the ECM can also be used to promote materials templating, which we demonstrate using BIND composed of a CsgA-A3 fusion produced in PHL628 cells. The A3 peptide was previously developed by phage display to bind silver and has been shown to control the templating of silver nanoparticles [25] . The wild-type CsgA biofilm did not appreciably template silver nanoparticles ( Fig. 3a ). In contrast, the A3-BIND biofilms show an enhanced ability to bind to growing silver nanoparticles from a solution of AgNO 3 , as shown by representative TEM images of incubated A3-BIND showing the assembly of nanoparticles throughout the nanofibres ( Fig. 3b,c ). These results are reproducible ( Supplementary Fig. 8 ) and demonstrate the utility of programmable biofilm matrices for the templating and organization of nanoparticles to form one-dimensional nanowires. The resulting nanoparticle-decorated nanofibres show a striking resemblance to naturally occurring metal-reducing extracellular fibres from Geobacter sulfurreducens , which have been shown to be electrically conductive [39] , suggesting that BIND-based biotemplating may be a viable strategy for the large-scale de novo production of conductive nanowires. Figure 3: Nanoparticle templating by BIND. Silver nanoparticles were templated by A3-BIND biofilms incubated in aqueous AgNO 3 . Representative TEM micrographs demonstrate that PHL628 Δ csgA cells producing wild-type CsgA ( a ) show no nanoparticle templating, whereas A3-BIND ( b ) templates nanoparticles after incubation in 147 mM AgNO 3 for 4 h. ( c ) A higher magnification of the Ag nanoparticles organized on A3-BIND nanofilaments is shown. All scale bars are 0.5 μm. Full size image Programmed BIND adhesion to 304L stainless steel To make BIND an efficient platform for developing interfacial materials, it will be critical to tune the nanofibre adhesion to specific abiotic surfaces. As an example of this capability, we tested the adhesion of E. coli cells displaying MBD to 304L stainless steel, the most versatile and widely used steel alloy. PHL628 cells producing the CsgA-MBD mutant were spotted onto 304L coupons ( Fig. 4a ), allowed to adhere for 48 h, and then vigorously washed by vortexing at a high setting in aqueous buffer to thoroughly remove nonspecifically bound cells. The spotted areas were analysed by SEM and showed that BIND composed of the CsgA-MBD fusion withstood the washing procedure ( Fig. 3b-d ), whereas the no CsgA or wild-type CsgA control cells were washed off the surface ( Supplementary Fig. 9 ). This result demonstrates that BIND programming using MBD is sufficient to impart adhesive function to biofilms that can withstand very rigorous washing conditions. The modularity of the BIND platform lends itself to a plug-and-play approach for the design of programmed biofilm adhesion for applications in bioremediation or chemical synthesis, where nonspecific biofilm growth is viewed as a disadvantage. This capability will be particularly useful in applications where patterned surfaces are used to spatially control biofilm formation [40] , or where it is desirable to localize biofilm growth to specific materials and resist detachment forces, as is often the case in industrial bioreactors [41] , [42] . 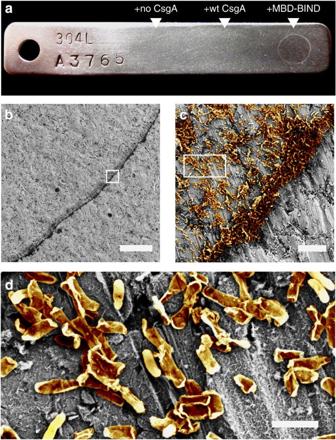Figure 4: BIND biofilms can be programmed to adhere to specific substrates. (a) Adhesion of PHL628 ΔcsgAcells producing no CsgA (left), wild-type CsgA (middle) and CsgA-MBD (right) was tested by spotting induced cultures onto a 304L steel coupon and incubating for 48 h at 4 °C. The ring formation is due to cells being drawn to the edges of the droplet during drying, known as the ‘coffee ring effect’. (b)The MBD-BIND biofilms were analysed by FE-SEM. Scale bar is 250 μm. (c) Magnification of the boxed area inbof a false-coloured FE-SEM showing MBD-BIND cells adhered to the 304L surface. Scale bar is 10 μm. (d) Magnification of the boxed area incof a false-coloured FE-SEM showing a zoomed-in view of the cell bodies. Because of the vigorous washing process, some of the cell bodies appear damaged. Scale bar is 2 μm. Figure 4: BIND biofilms can be programmed to adhere to specific substrates. ( a ) Adhesion of PHL628 Δ csgA cells producing no CsgA (left), wild-type CsgA (middle) and CsgA-MBD (right) was tested by spotting induced cultures onto a 304L steel coupon and incubating for 48 h at 4 °C. The ring formation is due to cells being drawn to the edges of the droplet during drying, known as the ‘coffee ring effect’. ( b )The MBD-BIND biofilms were analysed by FE-SEM. Scale bar is 250 μm. ( c ) Magnification of the boxed area in b of a false-coloured FE-SEM showing MBD-BIND cells adhered to the 304L surface. Scale bar is 10 μm. ( d ) Magnification of the boxed area in c of a false-coloured FE-SEM showing a zoomed-in view of the cell bodies. Because of the vigorous washing process, some of the cell bodies appear damaged. Scale bar is 2 μm. Full size image Covalent immobilization of proteins using BIND In addition to displaying short peptides, we reasoned that the utility of the BIND system would be greatly expanded if it could be used to display full proteins of arbitrary length and dimensions to programme the biofilm with artificial enzymatic, electron transport or sensing capabilities. We therefore created a two-component genetically encodable strategy ( Fig. 5a ) to covalently immobilize proteins onto the BIND network, using a previously developed split-adhesin system [28] in which a 13-amino-acid peptide (SpyTag) forms a highly specific and spontaneous isopeptide bond with a 15-kDa protein (SpyCatcher). The first component of our protein immobilization approach is an engineered SpyTag-functionalized BIND ECM and the second component is a SpyCatcher protein fused to another protein of interest. As our arbitrary test protein for ECM immobilization, we chose green fluorescent protein (GFP). SpyTag-BIND biofilms were grown on a glass substrate using PHL628 cells and formed characteristic curli nanofibre networks when either wild-type CsgA or CsgA-SpyTag were produced ( Fig. 5b–g ). We recombinantly produced GFP-SpyCatcher and a non-functional mutant [28] (GFP-SpyCatcher E77Q ) and applied cell lysates containing these proteins to SpyTag-BIND or wild-type CsgA biofilms. Analysis by epifluorescence microscopy revealed, as expected, that only the combination of biofilms composed of CsgA-SpyTag incubated with GFP-SpyCatcher resulted in covalent attachment ( Fig. 5h ). To further validate that the GFP-SpyCatcher is localized to the extracellular material and not to the cells, we analysed SpyTag-BIND+GFP-SpyCatcher samples using confocal microscopy and aligned the high-resolution fluorescence images with SEM micrographs of the same sample ( Supplementary Fig. 10a-c ). Regions that are fluorescent ( Supplementary Fig. 10d,e,g,h ) clearly correlate to regions that have a high density of ECM ( Supplementary Fig. 10e,f,h,i ). These results confirm that the SpyTag peptide can be fused to CsgA and maintain its functionality as a catalytic covalent immobilization tag after extracellular assembly into curli nanofibres. Furthermore, the use of unpurified cell lysate containing the GFP-SpyCatcher fusion protein demonstrates the robust binding specificity between the SpyTag-functionalized curli network and the SpyCatcher fusion protein, even in complex mixtures. This feature of BIND will be especially useful in the development of biocatalysts and biosensors, for the development of a facile and efficient enzyme immobilization process. 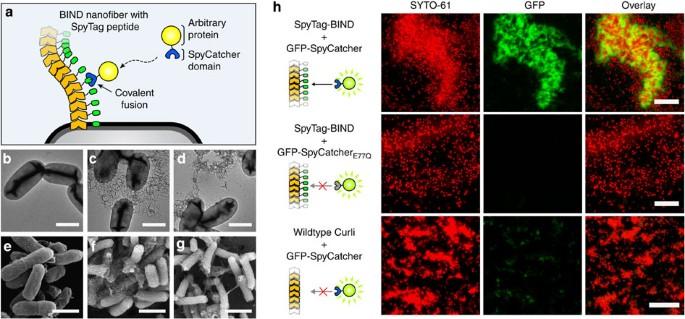Figure 5: Covalent immobilization of full-length proteins onto SpyTag-BIND biofilms. (a) The BIND immobilization strategy that uses an isopeptide bond-forming split-proteinS. pyogenesFbaB adhesin system28to covalently attach proteins fused to the SpyCatcher domain onto BIND biofilms displaying the 13-residue SpyTag. TEM and FE-SEM images, respectively, of PHL628 ΔcsgAstrains expressing no curli (b,e), wild-type CsgA (c,f) and the SpyTag-BIND biofilms (d,g); scale bars are 1 μm. (h) SpyTag-BIND biofilms were grown on PLL-modified glass substrates and then visualized with a nucleic-acid stain (SYTO61) followed by incubation with a cell lysate containing GFP-SpyCatcher fusion protein; scale bars are 25 μm. Epifluorescence microscopy of the biofilms reveals that only the proper combination of CsgA-SpyTag-BIND biofilms and GFP-SpyCatcher protein-containing cell lysate results in significant protein immobilization (top row). In contrast, SpyTag-BIND biofilms combined with a GFP-SpyCatcherE77Qprotein that has a key catalytic residue mutated in the SpyCatcher domain showed no immobilization (middle row). Wild-type CsgA biofilms combined with GFP-SpyCatcher also do now show significant immobilization. Figure 5: Covalent immobilization of full-length proteins onto SpyTag-BIND biofilms. ( a ) The BIND immobilization strategy that uses an isopeptide bond-forming split-protein S. pyogenes FbaB adhesin system [28] to covalently attach proteins fused to the SpyCatcher domain onto BIND biofilms displaying the 13-residue SpyTag. TEM and FE-SEM images, respectively, of PHL628 Δ csgA strains expressing no curli ( b , e ), wild-type CsgA ( c , f ) and the SpyTag-BIND biofilms ( d , g ); scale bars are 1 μm. ( h ) SpyTag-BIND biofilms were grown on PLL-modified glass substrates and then visualized with a nucleic-acid stain (SYTO61) followed by incubation with a cell lysate containing GFP-SpyCatcher fusion protein; scale bars are 25 μm. Epifluorescence microscopy of the biofilms reveals that only the proper combination of CsgA-SpyTag-BIND biofilms and GFP-SpyCatcher protein-containing cell lysate results in significant protein immobilization (top row). In contrast, SpyTag-BIND biofilms combined with a GFP-SpyCatcher E77Q protein that has a key catalytic residue mutated in the SpyCatcher domain showed no immobilization (middle row). Wild-type CsgA biofilms combined with GFP-SpyCatcher also do now show significant immobilization. Full size image BIND can be used to engineer multifunctional biofilms Previous research has shown that cross-seeding between even distantly related amyloid proteins can occur, resulting in composite nanofibres [43] . A key aspect of our BIND system is that by virtue of the random extracellular self-assembly of CsgA monomers, the simultaneous secretion of different CsgA fusions will result in a formation of a multifunctional biofilm surface. To demonstrate the generation of a biofilm ECM containing multiple artificially designed functions, we co-cultured PHL628 cells producing CsgA-FLAG and CsgA-SpyTag fusion proteins to produce a bifunctional BIND biofilm that can display the FLAG tag as well as immobilize GFP through the SpyTag-SpyCatcher system ( Fig. 6 ). Only the co-cultured sample is able to co-localize the GFP-SpyCatcher and a fluorescently labelled anti-FLAG antibody, as visualized by confocal microscopy ( Fig. 6 , bottom row). This capability of engineering multifunctional biofilms greatly increases the utility of our system for complex applications, which require any combination of adhesion, display, molecular templating or protein immobilization. 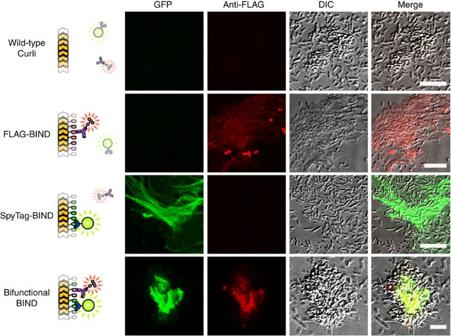Figure 6: BIND can be used to generate programmable multifunctional biofilms. Wild-type CsgA, FLAG-BIND, SpyTag-BIND and a co-culture of FLAG-BIND and SpyTag-BIND were all probed with GFP-SpyCatcher followed by anti-FLAG DyLight650-conjugated antibody. Confocal microscopy images for the GFP, DyLight650 and DIC (differential interference contrast) channels are shown. All scale bars are 5 μm. Figure 6: BIND can be used to generate programmable multifunctional biofilms. Wild-type CsgA, FLAG-BIND, SpyTag-BIND and a co-culture of FLAG-BIND and SpyTag-BIND were all probed with GFP-SpyCatcher followed by anti-FLAG DyLight650-conjugated antibody. Confocal microscopy images for the GFP, DyLight650 and DIC (differential interference contrast) channels are shown. All scale bars are 5 μm. Full size image Here we have demonstrated a strategy, BIND, for the rational molecular design of a microbial ECM component with the purpose of introducing new function into a biofilm. The biofilms of E. coli are partly composed of a functional amyloid nanofibre, curli, which plays a role in bacterial adhesion [44] , aggregation [43] and biofilm stability [37] , [45] . Our results show that the curli system in E. coli is capable of secreting a wide variety of chimeric CsgA-peptide constructs that can self-assemble into the ECM as amyloid nanofibres. The fused peptide domains are displayed in high density on the network surface and maintain their function even after assembly. The resulting nanofibre networks maintain their ability to encapsulate the cells and show morphological heterogeneity, with some variants exhibiting the tendency to form dense three-dimensional crypt-like structures or expansive fabric-like sheets ( Supplementary Fig. 11 ). Indeed, further exploration of the ability to control the three-dimensional morphology of curli-based nanostructures solely by altering the sequence of CsgA-peptide fusions seems warranted. We then selected three of these artificially designed biofilm materials to demonstrate that three distinct and diverse non-natural functions (silver nanoparticle templating, strong adhesion to steel surfaces and covalent protein immobilization) can be introduced modularly into E. coli biofilms based on the predetermined functions of various engineered peptide sequences. Our results show that biotemplating, substrate adhesion and protein immobilization can be readily programmed into a bacterial ECM. Importantly, this was accomplished without the need for system re-optimization, suggesting that other sequences can easily be incorporated into our system to access materials with a vast range of non-natural functions. In addition, a co-culture of cells harbouring different CsgA fusions resulted in a bifunctional biofilm, suggesting that the modular aspect of our platform can be used to engineer biofilms with a wide combination of desired functions. The BIND technology lends itself to the rapid development of interfacial nanomaterials with functions that can be drawn from the diverse repertoire of known natural and artificial peptides and proteins. These biofilm-based materials can be used in a wide range of environments that may or may not be conducive to cellular survival. In hospitable environments, the encapsulated cells of the biofilm may be induced to self-regenerate or heal the material over time, or remodel the material in response to environmental cues. In harsher environments, the highly robust amyloid matrix, once assembled, could persist beyond the lifetime of the cellular components as an acellular structure without the need for maintenance. In principle, our approach can be used to introduce new function to many other microbial biofilms with analogous functional amyloids (for example, Salmonella [46] , Pseudomonas [47] , Bacillus [48] spp.) to capitalize on the particular features of each wild-type strain. Given that the engineered bacteria proliferate rapidly and require no petroleum-derived raw building blocks in order to biosynthesize the external matrix, BIND may be useful as a scalable and green approach for fabricating customized interfacial materials across a wide range of size scales and environments. Recent work with synthetic gene circuits allows for the control of biofilm formation and dispersal dynamics through the engineering of global biofilm regulatory proteins [7] , [49] , [50] . Other work has paved the way for the patterning and control of curli composition [14] . By combining such biofilm control strategies with the ability to widely programme the functional properties of the ECM as we present here with BIND platform, we envision a merging of synthetic biology and materials science approaches. This would allow the development of large-scale programmable ‘living’ materials in which bacteria act as autonomous and self-replicating distributed molecular factories for the production of large-scale materials. In addition, engineered complex genetic logic gates could be used to switch on one or more defined BIND biofilms under specific environmental cues. This would potentially allow a single cell to encode for tens and possibly hundreds of different artificial BIND variants that could dynamically alter the bacterial ECM properties on demand. Cell strains and plasmids All cloning and protein production were performed in Mach1 (Life Technologies) and Rosetta cells (EMD Millipore), respectively. The csgA gene was isolated from E. coli K-12 genomic DNA and cloned into pBbE1a [51] , a ColE1 plasmid under control of the Trc promoter (Addgene). Peptide insert regions were either fully synthesized (Integrated DNA Technologies) or PCR-generated by overlap extension [52] . All cloning was performed using isothermal Gibson Assembly [53] and verified by DNA sequencing. The csgA deletion mutant LSR10 (MC4100, Δ csgA ) was a kind gift from the Chapman Laboratory. The csgA deletion mutant PHL628-ΔcsgA (MG1655 , malA-Kan ompR234 ΔcsgA ) was provided by the Hay Laboratory. All cell strains, plasmids and primers used in this study are fully provided in the Supplementary section ( Supplementary Tables 1, 2 and 3 ). Curli biofilm formation To produce curli, LSR10 cells or PHL628 cells were transformed with pBbE1a plasmids encoding for CsgA or CsgA-peptide fusions. As a negative control, cells were transformed with empty pBbE1a plasmid. The cells were then streaked or spotted onto YESCA-CR plates [54] , containing 10 g l −1 of casamino acids, 1 g l −1 of yeast extract and 20 g l −1 of agar. These plates were supplemented with 100 μg ml −1 of ampicillin, 0.5 mM of IPTG, 25 μg ml −1 of CRand 5 μg ml −1 of Brilliant Blue G250. The plates were then incubated for 48 h at 25 °C and then imaged to determine the extent of CR binding. For the spotted plates, the transformants were grown in YESCA liquid media supplemented with 100 μg ml −1 of ampicillin and 0.2 mM of IPTG for 48 h at 25 °C before spotting 20 μl onto YESCA-CR plates. SEM Curliated wild-type or BIND cell samples were either directly taken from induced YESCA cultures or scraped from YESCA-CR plates and resuspended in Millipore H 2 O. For SEM analysis, samples were applied to Nuclepore filters (0.22 μm pore size; GE Healthcare Bio-Sciences) under vacuum, washed with Millipore H 2 O and fixed with 2% glutaraldehyde+2% paraformaldehyde overnight at 4 °C, followed by fixation in 1% osmium tetroxide. The samples were then washed in Millipore H 2 O, dehydrated with an increasing ethanol step gradient, followed by a hexamethyldisilazane step gradient before gold sputtering and analysis on a Zeiss Supra55VP FE-SEM. TEM Curliated wild-type or BIND cell samples were either directly taken from induced YESCA liquid cultures or scraped from YESCA-CR plates and resuspended into Millipore H 2 O. For TEM analysis, 5 μl of the sample was spotted onto formvar-carbon grids (Electron Microscopy Sciences), washed with Millipore H 2 O and stained with 1% uranyl formate before analysis on a JEOL 1200 TEM. Whole-cell filtration ELISA To quantitatively detect the presence of extracellular CsgA as high-molecular-weight assemblies, an adapted whole-cell filtration ELISA protocol for detecting bacterial surface antigens was used [55] . BIND transformants were used to inoculate 3 ml YESCA liquid cultures supplemented with 50 μg ml −1 of carbenicillin, grown to mid-log phase and induced with 0.25 mM of IPTG. The induced cells were incubated at 25 °C for 48 h before analysis. The cultures were subsequently placed on ice and all were diluted to an OD 600 of 0.1 using Tris-buffered saline (TBS). Sodium azide of 0.1% was added to inhibit cell metabolism. To a Multiscreen-GV 96-well filter plate (0.22 μm pore size; EMD Millipore), 25 μl of the diluted culture was added and washed three times in wash buffer (TBS+0.1% Tween-20+0.1% NaN 3 ) and incubated in 200 μl of Blocking Buffer (wash buffer supplemented with 1% bovine serum albumin and 0.01% H 2 O 2 ) for 1 h at 37 °C. The H 2 O 2 is needed to inactivate endogenous cellular peroxidases [55] . The samples were then washed three times in wash buffer, incubated with anti-CsgA primary antibody [8] diluted to 1:10,000 in wash buffer for 1 h at 25 °C, washed three more times in wash buffer and then incubated with goat anti-rabbit HRP-conjugated secondary antibody (Thermo Fisher Scientific) diluted to 1:5,000 in wash buffer for 1 h at 25 °C. After a final washing step three times in wash buffer, the samples were processed using the Ultra-TMB (3,3′,5,5′-tetramethylbenzidine) ELISA substrate (Thermo Fisher Scientific), adding 100 μl per well. After incubation at room temperature for 5 min, the reaction was terminated by the addition of 50 μl of 2 M H 2 SO 4 . Exactly 100 μl of this reaction was transferred to a flat-bottom 96-well plate and analysed on a BioTek Synergy H1 Multi-Mode Plate Reader, measuring the absorbance at 450 nm and a reference wavelength of 650 nm. MBD-BIND binding to 304L stainless steel coupons Steel alloy 304L coupons (Alabama Specialty Products, Inc.) were cleaned with fine-grit sandpaper, acetone, Millipore water, sonicated in 1 M NaOH for 1 h at 80 °C, washed again with Millipore water and finally rinsed with acetone before air-drying. PHL628- ΔcsgA transformants were grown in YESCA media as described above and induced by adding 0.5 mM IPTG and 3% DMSO for 48 h at 25 °C, 150 r.p.m. Cell cultures were normalized to an OD 600 of 1 and 20 μl was spotted onto a 304L coupon. The spotted coupon was placed in a sterile Petri dish and placed in 4 °C to allow attachment and minimize evaporation. After 48 h, the coupons were rinsed briefly with PBST, placed in a tube filled with PBST, and vigorously vortexed three times for 30 s. The coupons were then fixed and imaged using SEM according to the protocols described above. Silver nanoparticle templating PHL628- ΔcsgA cells were transformed with wild-type CsgA, and CsgA-A3-expressing plasmids and induced with 0.2 mM IPTG in YESCA broth containing 100 μg ml −1 carbenicillin for 48 h. The cells and curli were isolated by pelleting and then resuspended in PBS+calcium and magnesium (CM). Nickle-formvar/carbon TEM grids were floated on drops of these resuspended samples, washed two times with PBS+CM, three times with Millipore H 2 O and then incubated on a drop containing 147 mM AgNO 3 for 4 h. The grids were then washed three times with mpH 2 O and negatively stained and analysed by TEM as described above. Incubation with lower amounts of AgNO 3 for longer periods of time resulted in substantial cell lysis, complicating the analysis. Biofilm fluorescence microscopy imaging PHL628-Δ csgA cells transformed with control, wild-type CsgA and CsgA-SpyTag-expressing plasmids were grown up in 20 ml YESCA broth containing 100 μg ml −1 ampicillin at 30 °C until an OD of 0.6. Plasma-activated and PLL-functionalized coverslips were placed into the cultures and curli expression and biofilm formation were induced by adding 0.5 mM IPTG and 3% DMSO. Cultures were grown at 25 °C and 150 r.p.m. for 48 h. Slides were removed from the cultures and washed 3 × 20 min in wash buffer (1 × PBS+0.5% Tween-20), shaking at 150 r.p.m. After the washes, 0.5 ml of 1 mg ml −1 GFP-SpyCatcher- or GFP-SpyCatcher(E77Q)-containing cell lysate solution (in PBS+1% BSA+0.5% Tween) was added to slides. The biofilms were incubated for 1 h and then washed 2 × 20 min with wash buffer. The samples were then stained with SYTO-61 (10 μM) for 20 min and washed with wash buffer 2x 15 min shaking at 150 r.p.m. Slides were then imaged in epifluorescence mode on a Leica TIRF DM16000B at × 60 and × 100. For the multifunctional BIND experiments, cells at an initial OD 600 of 2.5 were cultured in MatTek glass-bottom dishes for 72 h under inducing conditions (YESCA/0.5 mM IPTG/100 ng ml −1 carbenicillin/3% DMSO). The biofilms were then washed 3 × 10 min in PBST, blocked with 1% BSA in PBST for 1 h and incubated with GFP-SpyCatcher-containing clarified cell lysate for 1 h. The dishes were then extensively washed with 0.1% BSA+PBST under gentle shaking before incubation with an anti-FLAG DyLight 680 antibody (Pierce) for 1 h. The samples were washed as before with 0.1% BSA+PBST, fixed with 2% glutaraldehyde+2% paraformaldehyde in 0.1 M sodium cacodylate buffer for 15 min and then incubated in PBS+10 mM glycine overnight at 4 °C to eliminate autofluorescence. All multifunctional BIND samples were analysed on Leica SP5 X MP Inverted Confocal Microscope with identical laser power and detector integration settings. CR birefringence analysis Spotted LSR10 transformants grown for 48–72 h at 25 °C on YESCA-CR plates were scraped and spread onto glass slides in a drop of PBS. The samples were covered with a coverslip and analysed on a Zeiss Axio Observer Z1 microscope fitted with polarization filters. Contrast adjustment and background subtraction were performed using ImageJ [56] . Purification of curli-enriched pellets The purification method for MALDI analysis of curli samples was adapted from Römling et al . [57] LSR10 transformants were spread onto YESCA plates supplemented with 50 μg ml −1 of carbenicillin and 0.5 mM of IPTG. After 72 h growth at 25 °C, the cells were harvested from the plates and resuspended in 2.5 ml of TBS. Curli fibres were sheared from the cells by sonication using a Qsonica Q700 Sonicator at 15% power with 30 s pulse/2 min rest/3 min total processing. The cells were then pelleted at 3,500 r.p.m. for 20 min. The supernatant was collected and incubated in 1% SDS+250 mM NaOH for 1 h with shaking at room temperature. The SDS-insoluble material was pelleted by ultracentrifugation in a Beckman Coulter Optima XPN Preparatory Ultracentrifuge (Beckman Coulter) at 120,000 g for 30 min. The resulting insoluble pellet was resuspended in 5 ml of ultrapure water and pelleted again by ultracentrifugation. This washing process was then repeated one more time. The final curli-enriched pellet was resuspended in 100 μl of Millipore water and lyophilized. MALDI analysis of dissolved SDS-insoluble extracellular fractions To confirm that BIND biofilms contain full-length CsgA fusion proteins instead of proteolysed fragments, MALDI analysis was performed on dissolved curli-enriched pellets. The lyophilized curli-enriched pellet was resuspended in 50 μl of HFIP to dissolve the amyloid curli fibres into monomers. HFIP is commonly used to dissolve amyloids in lieu of formic acid to prevent acid hydrolysis of protein samples [58] . After incubation for 1 h in HFIP, the solvent was evaporated by a stream of nitrogen. The HFIP-treated samples were then redissolved in a minimal volume of 1:1 acetonitrile-H 2 O with 0.1% trifluoroacetic acid (TFA) and applied to the sample plate using the sandwich method with sinapinic acid (Thermo Fisher Scientific) as the MALDI matrix [59] . The dried samples were then analysed on a Bruker ultrafleXtreme MALDI-TOF/TOF in linear mode. All spectra were calibrated using Bruker Protein Calibration Standards I (Bruker Biosciences Corp.). Immunogold TEM For anti-FLAG immunogold labelling of the BIND cells displaying the FLAG tag, the cells were first adhered to nickel TEM grids (Electron Microscopy Sciences) as described above. Then, the grids were washed 3 × in blocking buffer (PBS+1% BSA), floated face-down on a drop containing a 1:1,000 dilution of primary anti-FLAG murine antibody (Sigma-Aldrich) in PBS for 30 min, washed in blocking buffer again, and then floated on a drop of 1:1,000 diluted anti-mouse 15 nm gold-conjugated antibody (Ted Pella, Inc) for 30 min. After a final 3x wash in PBS and a wash in Millipore H 2 O, the grids were stained with 1% uranyl formate (Electron Microscopy Sciences) for 15 s and imaged on a JEOL 1200 TEM. How to cite this article : Nguyen, P. Q. et al . Programmable biofilm-based materials from engineered curli nanofibres. Nat. Commun. 5:4945 doi: 10.1038/ncomms5945 (2014).